Phase transitions in natural C-O-H-N-S fluid inclusions - implications for gas mixtures and the behavior of solid H2S at low temperatures C–O–H–N–S-bearing fluids are known as one of the most challenging geochemical systems due to scarcity of available experimental data. H 2 S-rich fluid systems were recognized in a wide array of world-class mineral deposits and hydrocarbon reservoirs. Here we report on a nature of low-temperature ( T ≥ −192 °C) phase transitions observed in natural CH 4 –H 2 S–CO 2 –N 2 –H 2 O fluid inclusions, which are modeled as closed thermodynamic systems and thus serve as natural micro-laboratories representative of the C–O–H–N–S system. For the first time, we document solid–solid H 2 S (α ↔ β ↔ γ) transitions, complex clathrates and structural transformations of solid state H 2 S in natural inclusion gas mixtures. The new data on Raman spectroscopic features and a complete sequence of phase transition temperatures in the gas mixtures contribute to scientific advancements in fluid geochemistry. Enhanced understanding of the phase equilibria in the C–O–H–N–S system is a prerequisite for conscientious estimation of P-T-V-X properties, necessary to model the geologic evolution of hydrocarbon and mineral systems. Our findings are a driver for the future research expeditions to extraterrestrial H 2 S-rich planetary systems owing to their low temperature environments. Hydrogen sulfide (H 2 S) is a natural gas of organic or inorganic origin. At shallow crustal levels, it is produced in anaerobic environments by degradation of biomass [1] . As biological mediator H 2 S plays an important role in the global sulfur cycle and the evolution of life on Earth [2] . Recent research has shown that H 2 S-bearing gaseous fluid inclusions carry information imperative to understanding the building blocks of early Archean life [3] . Inorganic H 2 S is a common constituent in volcanic gases [4] , active black smoker vents [5] , and carbonate-hosted hydrocarbon reservoirs [6] , [7] , [8] . Dissolved in water, H 2 S or its dissociation products are indispensable for the formation of precious [9] and base metal deposits [10] . Recent discoveries of H 2 S-ice on Uranus and Neptune at temperatures ranging between −220 [11] and −153.7 °C [12] , [13] , reveal that the low-temperature conditions, which this study focuses on, find clear analogs in the Solar System. Hence, the processes investigated here are of essential importance for understanding the natural terrestrial as well as extraterrestrial environments. In materials science, H 2 S is utilized to synthesize superconductive materials in the form of sulfur hydrides, e.g., H 3 S, which displays superconductive properties at transition pressure of 155 GPa and temperature of −70.15 °C [14] . This finding was an important breakthrough in the development of room-temperature CSH 8 superconductor [15] . Determining fluid properties and understanding the phase relations in the P-T-V m space are paramount in fluid geochemistry and geological sciences [16] , [17] . Mineral-hosted natural fluid inclusions, which preserve fluids from various geological records in micrometer-scale cavities, are a powerful tool to characterize fluid properties. Fluid inclusions are modeled as “closed” systems, meaning that they permit heat exchange, whereas their molar volumes ( V m ) and compositions ( X i ) remain constant throughout the geological evolution. Consequently, the P–T conditions of fluid inclusion trapping are deduced from the isochoric trajectories [18] , which are constructed from bulk V m - X i parameters. Microthermometry allows observation of fluid inclusion phase transition temperatures, which can be converted into V m and X i by applying equations of state (EoS) or/and quantitative phase diagrams [19] . Laser Raman spectroscopy allows to determine molecular compositions of complex C–O–H–N–S inclusion gas mixtures [8] , [10] , [20] , [21] , [22] , [23] . Combined microthermometric and Raman spectroscopic analyses coupled with phase diagrams/EoS provide means to reconstruct the spatial and temporal P–T evolution in mineralizing systems [10] , [24] and gas reservoirs [8] , [21] , [22] , [25] . The latter are often characterized by multiple episodes of coinciding mineralization and gas/oil re-charge. P–T estimates in such systems rely on the construction of isochores for gaseous and/or aqueous fluid inclusions [26] . This is challenging for CH 4 –H 2 S–CO 2 –N 2 inclusions, which contain elevated H 2 S concentrations [27] , [28] since the properties of the C–O–H–N–S gas mixtures are poorly constrained by experimental and thermodynamic data [29] . Natural H 2 S-bearing fluid inclusions representing binary CH 4 –H 2 S and CO 2 –H 2 S systems have been characterized in terms of molecular compositions and phase changes [30] as phase equilibria of these two systems are well constrained by experimental studies [31] , [32] , [33] , [34] , [35] . In contrast, experimental data for ternary system CH 4 –CO 2 –H 2 S are scarce and cover only very limited P–T–X ranges with a focus on the near-critical region of the system [36] , [37] , [38] . An influence of subordinate amounts of CO 2 on phase equilibria in the CH 4 –H 2 S system in the low-temperature region remains unclear [30] , [32] . Experimental studies on purified H 2 S gas have shown that three structurally distinct solid H 2 S phases (I-α, II-β, and III-γ) form at low temperatures below −85.5 °C [39] . Crystal symmetry of the H 2 S-γ phase, which forms at the lowest temperatures below −169.6 °C, has been under debate [39] , [40] , [41] , [42] . Laser Raman spectroscopy is one of the most effective techniques in distinguishing structurally distinct solid H 2 S molecules [39] , [42] , [43] . The structure of H 2 S solid phases and solid–solid phase transitions have not been recognized in natural fluid inclusions up to date. In this study, we investigate fluorite-hosted H 2 S-bearing fluid inclusions representing the natural CH 4 –H 2 S–CO 2 –N 2 –H 2 O system. We use combined microthermometric and Raman spectroscopic analyses to record the complete sequence of phase transition temperatures as well as compositions and spectral features of individual phases at low temperatures. Fluid inclusion assemblages Fluid inclusions were analyzed in line with the classic concept of a fluid inclusion assemblage (FIA) [44] . Both selected FIA’s (Fig. 1 ), consisting of low-density gas-rich (V) and aqueous 2-phase inclusions (L + V), evidence precipitation of fluorite in the presence of methane, inorganic gases (H 2 S, CO 2 , N 2 ) as well as small proportions of a high salinity brine. 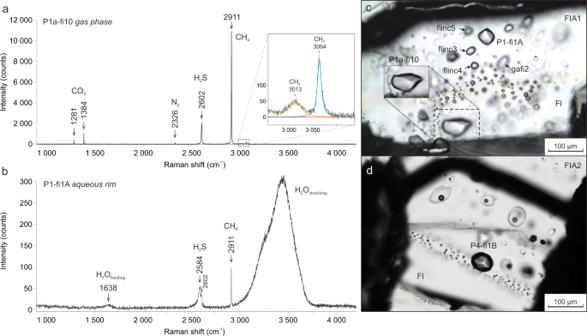Fig. 1: Fluid inclusion assemblages (FIA’s) at room temperature. aRaman spectrum of the gas phase in the gas-rich fluid inclusions shows sharp peaks typical of the gas mixture: CH4(2911 cm−1), H2S (2602 cm−1), CO2Fermi diad (1281 cm−1, 1384 cm−1), and N2(2326 cm−1), representing symmetric stretching vibrations (ν1) of the gas molecules. Weak intensity broad peak at 3013 cm−1is attributed to the triply degenerate anti-symmetric C–H stretching of CH4gas, whereas a weak 2ν2overtone at 3064 cm−1is assigned to the doubly degenerateν2mode vibration of CH4gas49.bRaman spectrum of the aqueous phase rim surrounding the gas phase. The broad Raman peak between 3000 and 3700 cm−1, and weak peak at 1638 cm−1correspond to stretching and bending vibrations in H2O, respectively. The low-intensity Raman band at 2584 cm−1is assigned to H2S dissolved in water.c,dMicrophotographs of analyzed CH4–H2S–CO2–N2–H2O fluid inclusions in FIA1 and FIA2 hosted in fluorite (Fl). The molecular compositions of gas phases in the gas-rich inclusions are shown in Table 1 , Supplementary Table 1 , and Source Data. Fig. 1: Fluid inclusion assemblages (FIA’s) at room temperature. a Raman spectrum of the gas phase in the gas-rich fluid inclusions shows sharp peaks typical of the gas mixture: CH 4 (2911 cm − 1 ), H 2 S (2602 cm − 1 ), CO 2 Fermi diad (1281 cm − 1 , 1384 cm − 1 ), and N 2 (2326 cm − 1 ), representing symmetric stretching vibrations ( ν 1 ) of the gas molecules. Weak intensity broad peak at 3013 cm − 1 is attributed to the triply degenerate anti-symmetric C–H stretching of CH 4 gas, whereas a weak 2 ν 2 overtone at 3064 cm − 1 is assigned to the doubly degenerate ν 2 mode vibration of CH 4 gas [49] . b Raman spectrum of the aqueous phase rim surrounding the gas phase. The broad Raman peak between 3000 and 3700 cm − 1 , and weak peak at 1638 cm − 1 correspond to stretching and bending vibrations in H 2 O, respectively. The low-intensity Raman band at 2584 cm − 1 is assigned to H 2 S dissolved in water. c , d Microphotographs of analyzed CH 4 –H 2 S–CO 2 –N 2 –H 2 O fluid inclusions in FIA1 and FIA2 hosted in fluorite (Fl). Full size image Table 1 Microthermometry data and molecular compositions of fluorite-hosted CH 4 –H 2 S–CO 2 –N 2 –H 2 O fluid inclusions from two fluid inclusion assemblages (FIA’s). Full size table The two biggest gas-rich inclusions (P1-fi1A, P1a-fi10) in FIA1 contain a visible aqueous film surrounding the gas phase, whereas in the smaller inclusions the aqueous phase is optically invisible. The bimodal distribution, lack of intermediate aqueous fluid/gas ratios, and gas-saturation (in respect of CH 4 , CO 2 , and H 2 S) of the vapor phases of co-existing aqueous brine inclusions imply contemporaneous trapping of immiscible fluids. Fluorite growth from aqueous brine was obstructed by the gas bubbles, which were wet by traces of the aqueous medium during the fluid entrapment. Thus, it is very unlikely to form water-free, pure gas inclusions in such hydrothermal systems. When heating the inclusions to temperatures up to 170 °C, Raman spectroscopic analyses of the homogenized inclusion fluid [45] point to the presence of 3 mol% H 2 O in all gas-rich inclusions (Table 1 , Supplementary Fig. 1 and Source Data). The volume fractions of the aqueous phase ( φ H2O ) [46] in two inclusions with optically visible aqueous rim, indicate very similar water contents of 2.2 and 3.5 wt.%. The water vapor or dissolved H 2 O was not detected in the gas phase of the gas-rich inclusions at room temperature (Fig. 1a ). The gas compositions of six measured inclusions within a single FIA1 (Table 1 ) are very similar as indicated by very low standard deviation values (σ < 0.02). Median gas compositions for FIA1 are 59 mol% CH 4 , 24 mol% H 2 S, 10 mol% CO 2 , 3 mol% N 2 , whereas FIA2 shows a slightly higher H 2 S content of 27 mol% (Table 1 and Fig. 1 ). The aqueous rims of the gas-rich inclusions are H 2 S saturated as indicated by the broader Raman peak at 2584 cm − 1 , which is typical of H 2 S dissolved in water at room temperature (Fig. 1b ). The origin of low-intensity gas peaks in the latter spectrum is ambiguous, they may be derived from gas species dissolved in water and/or may constitute peak overlaps from a much larger gas phase. The steep band between 3000 and 3700 cm − 1 , corresponding to the stretching vibrations of H 2 O, confirms the high salinity [47] of the aqueous solution coating the gas inclusion (Fig. 1b ). Low-temperature phase transitions—freezing runs Eight phase transitions were recognized in the studied gas-rich inclusions during freezing (Fig. 2a–i ) and heating runs (Fig. 2j–p ). 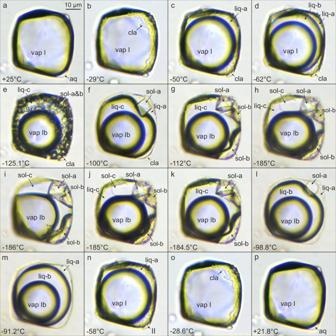Fig. 2: Transmitted light microphotographs of phase transitions in CH4–H2S–CO2–N2–H2O fluid inclusion (no. P1-fi1A) during freezing and heating runs. aOne-phase gas inclusion (vap I) at room temperature.bClathrate (cla) formation as a result of the aqueous rim (aq) wetting the gas inclusion.cExsolution of liquid H2S phase (liq-a).dUnmixing of liquid CH4-CO2phase (liq-b).eInstantaneous and simultaneous crystallization of liquid H2S and liquid CO2into a fine-grained ice mass.fNucleation of an octahedral CO2crystal (sol-a) in the presence of liquid H2S (liq-a) produced by heating-freezing cycling run.gNucleation of two “blobby” H2S solids (sol-b) in the presence of liquid CH4(liq-c), by applying cycling technique.hContinuous solidification of methane with visible solid/liquid methane (sol-c/liq-c) phase boundary.iCo-existence of three solid phases: CH4(sol-c), H2S (sol-b), CO2(sol-a) and CH4-N2gas phase (vap Ib).j,kContinuous liquefaction of solid CH4(sol-c) until completion at −184.5°C.lRounded CO2solid (sol-a) in the presence of liquid H2S (liq-a) after H2S solid melted at −98.8 °C.m,nPost-CO2solid melting at −91.2 °C, continuous vaporization of liquid CH4-CO2phase (liq-b), which is finalized by partial homogenization to a vapor phase (vap I).oVaporization of liquid H2S (liq-a) finalized by total homogenization to a vapor phase (vap I) at −28.6 °C.pMelting of clathrate (cla) at +21.8 °C. Symbols and abbreviations: vap-gas phases: vap I: CH4–H2S–CO2–N2, vap Ib: CH4–N2; cla-clathrate; liq-liquid phases: liq-a: H2S, liq-b: CH4–CO2, liq-c: CH4; sol-solid phases: sol-a: CO2, sol-b: H2S, sol-c: CH4; aq-aqueous solution. The complete temperature sequence of the phase changes is shown in Table 1 and Supplementary Table 2 . Two gas-rich inclusions P1-fi1A and P4-fi1B (hereinafter labeled inclusion A and B) of different molecular compositions (Table 1 ) were used to document in detail the phase transition sequences (Figs. 2 and 3 ). Fig. 2: Transmitted light microphotographs of phase transitions in CH 4 –H 2 S–CO 2 –N 2 –H 2 O fluid inclusion (no. P1-fi1A) during freezing and heating runs. a One-phase gas inclusion (vap I) at room temperature. b Clathrate (cla) formation as a result of the aqueous rim (aq) wetting the gas inclusion. c Exsolution of liquid H 2 S phase (liq-a). d Unmixing of liquid CH 4 -CO 2 phase (liq-b). e Instantaneous and simultaneous crystallization of liquid H 2 S and liquid CO 2 into a fine-grained ice mass. f Nucleation of an octahedral CO 2 crystal (sol-a) in the presence of liquid H 2 S (liq-a) produced by heating-freezing cycling run. g Nucleation of two “blobby” H 2 S solids (sol-b) in the presence of liquid CH 4 (liq-c), by applying cycling technique. h Continuous solidification of methane with visible solid/liquid methane (sol-c/liq-c) phase boundary. i Co-existence of three solid phases: CH 4 (sol-c), H 2 S (sol-b), CO 2 (sol-a) and CH 4 -N 2 gas phase (vap Ib). j , k Continuous liquefaction of solid CH 4 (sol-c) until completion at −184.5°C. l Rounded CO 2 solid (sol-a) in the presence of liquid H 2 S (liq-a) after H 2 S solid melted at −98.8 °C. m , n Post-CO 2 solid melting at −91.2 °C, continuous vaporization of liquid CH 4 -CO 2 phase (liq-b), which is finalized by partial homogenization to a vapor phase (vap I). o Vaporization of liquid H 2 S (liq-a) finalized by total homogenization to a vapor phase (vap I) at −28.6 °C. p Melting of clathrate (cla) at +21.8 °C. Symbols and abbreviations: vap-gas phases: vap I: CH 4 –H 2 S–CO 2 –N 2 , vap Ib: CH 4 –N 2 ; cla-clathrate; liq-liquid phases: liq-a: H 2 S, liq-b: CH 4 –CO 2 , liq-c: CH 4 ; sol-solid phases: sol-a: CO 2 , sol-b: H 2 S, sol-c: CH 4 ; aq-aqueous solution. Full size image Fig. 3: Microphotographs of phase transitions in CH 4 –H 2 S–CO 2 –N 2 –H 2 O fluid inclusion (no. P4-fi1B) in the temperature range between +25 and −190 °C, PPL, reflected light. a One-phase gas inclusion (vap-I) at room temperature. b Formation of clathrate (cla) at the fluid inclusion corners coated by an aqueous solution. c Exsolution of liquid H 2 S phase (liq-a). d Advanced stage of unmixing of liquid CH 4 –CO 2 phase (liq-b). e , f Instantaneous and simultaneous crystallization of liquid H 2 S and liquid CO 2 . g Nucleation of solid octahedral CO 2 crystal (sol-a) in the presence of liquid H 2 S (liq-a) by applying the cycling technique. h Nucleation of a large, oval H 2 S solid (H 2 S-α) via applying the cycling technique. i , j Co-existence of polycrystalline solid H 2 S (H 2 S-γ), solid CO 2 octahedral crystal (sol-a), solid CH 4 (sol-c), clathrate (cla) and CH 4 -N 2 gas phase (vap-Ib), a prismatic H 2 S-γ crystal is tagged with a white arrow. k , l Appearance of solid H 2 S after γ → β phase transformation, visible is structure change from ordered polycrystalline to disordered “blobby” during the heating run. Symbols and abbreviations: vap-gas phases: I: CH 4 -H 2 S-CO 2 -N 2 , Ib: CH 4 -N 2 ; cla-clathrate; liq-liquid phases: liq-a: H 2 S, liq-b: CH 4 –CO 2 , liq-c: CH 4 ; sol-solid phases: sol-a: CO 2 , H 2 S-α,β,γ: H 2 S, sol-c: CH 4 ; F-freezing run, C-cycling run, H-heating run. Green crosses mark several of Raman measurement points (see also Fig. 6 ). Full size image When cooling the inclusion to temperatures from −17 to −28.7 °C, the first solid phase that nucleates at the corners of the inclusion cavities is H 2 S-rich clathrate (Figs. 2 b and 3b ), which is manifested by two Raman bands at 2593 and 2604 cm − 1 (Fig. 4 ). In inclusions, containing a visible water film, the formation of H 2 S–CH 4 –CO 2 –N 2 clathrates is observed (Fig. 4 ). Raman peaks of 1276 and 1380 cm − 1 are typical for CO 2 -clathrate, bands at 2903 and 2913 cm − 1 are assigned to CH 4 -clathrate, whereas peak splitting to 2324 and 2323 cm − 1 is attributed to N 2 -gas hydrate [48] (Fig. 4a ). Fig. 4: Raman spectrum of natural clathrate in CH 4 -H 2 S-CO 2 -N 2 -H 2 O fluid inclusion (no. P1a-fi10) at −39 °C. An individual measurement records complex clathrate phase/s containing H 2 S, CH 4 and minor CO 2 , N 2 molecules. Additional Raman peaks at 3049 and 3121 cm − 1 , present in the O-H stretching spectral region, are assigned to a molecular vibration of CH 4 occluded in the hydrate lattice [49] and ice, respectively. a The inset shows low-intensity Raman bands corresponding to N–N stretching vibrations in N 2 -gas hydrate [48] and air N 2 . b Microphotograph of the analyzed clathrate solid in gas-rich inclusion. Symbols: vap-CH 4 –H 2 S–CO 2 –N 2 gas phase, cla-measured clathrate phase, liq-a-liquid H 2 S phase, the measurement point is marked with a green cross. The spectrum was acquired with 100% laser power. Full size image During further cooling below −29.9 °C/−32.6 °C (inclusions A/B) the H 2 S–CH 4 –CO 2 –N 2 gas phase begins to shrink due to volume reduction (Figs. 2c and 3c ) and partial separation of H 2 S-rich liquid. At temperatures of −58.6 °C/−58.5 °C (A/B) CH 4 -rich liquid starts to separate from the gas phase (Fig. 2d ). The presence of H 2 S- and CH 4 -rich liquids is indicated by the broadening and shift of the Raman bands to 2593 and 2908 cm − 1 , respectively. Raman analyses of the three resulting phases reveal that H 2 S-rich liquid partitions into the outermost phase, liquid CH 4 –CO 2 into the middle phase, whilst CH 4 –N 2 gases remain in the innermost bubble (Fig. 3d ). At −100 °C, vibrational bands of CH 4 –N 2 gases from the innermost phase show a shift to higher wavenumbers (2915 cm − 1 , 2328 cm − 1 ) compared with the gas phase at room temperature (2911 cm − 1 , 2326 cm − 1 ) (Fig. 5 ). Similar peak shifts are observed for CO 2 and H 2 S in the middle and the outermost phases, respectively. Fig. 5: Raman spectra of symmetric stretching (ν 1 ) region of CH 4 gas in a natural CH 4 –H 2 S–CO 2 –N 2 –H 2 O fluid inclusion gas mixture (no. P1-fi1A) at low temperatures. a – e Microphotographs of measured individual phases in analyzed gas-rich inclusion. f Sequence of Raman spectra showing that with decreasing temperature Raman peak positions of the exsolved liquid and gas methane shift to lower and higher wavenumbers, respectively. This is a result of relative density increase/decrease during differential partitioning between co-existing phases. The FWHM of the Raman peaks also decrease with decreasing temperatures. Symbols: I: CH 4 –H 2 S–CO 2 –N 2 gas, Ib: CH 4 –N 2 gas, II-clathrate, III-liquid phases: IIIa: H 2 S, IIIb: CH 4 –CO 2 , IIIc: CH 4 , IV-solid phases: IVa: CO 2 , IVα,γ: H 2 S, IVc: CH 4 , measurement points of different phases are marked with large and small crosses. Full size image At temperatures of −125.1 °C/−117.4 °C (A/B) both H 2 S and CO 2 simultaneously freeze and form a fine-grained mass of bright white (CO 2 ) and yellow-greenish solids (H 2 S-α) of high reflectance (Figs. 2e and 3e, f ). In order to investigate the composition and phase behavior of the nucleated solids a cycling heating/freezing method is applied [44] . After melting of solid H 2 S, the inclusion is heated further on until only one CO 2 crystal remains. Subsequent rapid cooling results in crystallization of a pure octahedral CO 2 crystal at −100 °C (Figs. 2f and 3g ), which shows Raman peaks at 1280 and 1384 cm − 1 . When cooling the inclusion to about −112 °C numerous oval solids of H 2 S-α crystallize. Applying the cycling heating/freezing procedure on H 2 S-α is difficult due to the very unstable “jelly-like” behavior of solids and rapid melting of the last solid upon approaching the final T m (H 2 S-α). However, when using slow heating rates (4 °C/min) until only some solids remain in the inclusion and then keeping the temperature constant for several minutes, involuntary re-organization of the leftover solids and formation of a single H 2 S-α solid phase is observed (Figs. 3 h and 5d ). At −110 °C solid H 2 S-α shows a single peak at 2558 cm − 1 (Fig. 6h ). Below −184 °C solidification of CH 4 commences (Fig. 2h, i ) and is completed at about −185.3 °C/−186.3 °C (A/B). The resulting CH 4 solid is characterized by a broad band at a vibrational frequency of 2904.5 cm − 1 . At −190 °C, Raman peaks of CH 4 and N 2 in the remaining squeezed gas phase are shifted towards the highest wavenumbers of 2917 and 2329 cm − 1 , respectively. Fig. 6: Raman spectra of the stretching region of H 2 S in a natural CH 4 –H 2 S–CO 2 –N 2 –H 2 O fluid inclusion (no. P4-fi1B) at low temperatures. A density-related shift in Raman peak positions to lower wavenumbers with decreasing temperature is observed for different physical states of H 2 S. The measurement points (a, d, h, k, i) are indicated by green crosses in the Fig. 3 . The solid H 2 S (γ ↔ β) phase transition is marked by intensity decrease of the characteristic peak of the β-phase and the progressive emergence of the sharp γ-phase peak at the lower wavenumber (2523 cm − 1 ) and its subsequent intensity increase. The solid H 2 S (γ ↔ β) phase transition was recorded during real-time measurements. Full size image The last optically visible phase change is structural re-configuration of H 2 S at about −191 °C. Smooth solids rearrange into very fine-grained polycrystalline aggregates (Fig. 3i, j ) over a prolonged period of time, meaning the transition is not instantaneous but requires a few minutes of maintaining the temperature constant. Notable is a prismatic H 2 S-γ crystal, tagged with white arrow in Fig. 3i , visible among the fine-grained crystals. This behavior marks the solid H 2 S (β → γ) transition, which actually commences at a higher temperature, however, it is not instantly visible under the optical microscope. The median temperature range for the H 2 S (β → γ) transition is between −175.1 and −176.1 °C, which gives an overall median of −175.6 °C and σ = 1.27 (Supplementary Table 2 ). The transformation to H 2 S-γ in the studied inclusion is reflected by the appearance of six characteristic peaks at the following wavenumbers: 2523, 2541, 2545, 2547, 2552, and 2556 cm − 1 (Figs. 6 and 7 ). The lower intensity five peaks on the high-frequency side of the Raman spectrum (Fig. 7 ) develop in an expense of the major H 2 S-β peak by decrease in its intensity (Fig. 6 ). These results are reproducible as H 2 S (γ ↔ β) transitions have been observed multiple times during real-time Raman spectroscopic analyses (Supplementary Table 2 ). Fig. 7: Raman spectrum of solid H 2 S-γ in a natural CH 4 –H 2 S–CO 2 –N 2 –H 2 O fluid inclusion (no. P4-fi1B). Six characteristic peaks are observed in the H–S spectral region at −191 °C. Five overlapping peaks have been deconvolved into separate bands and fitted using the Gaussian–Lorentzian peak-fitting function. The spectrum was acquired with 100% laser power. Full size image Low-temperature phase transitions—heating runs When heating the inclusion from −192 °C, eutectic melting of solid CH 4 is observed at about −185.5 °C until the final T m of −184.5 °C/−185 °C (A/B) is reached (Fig. 2j-k ). At about −168.1 °C (B), a rapid decrease in a band number of the H 2 S solid in the Raman spectrum is observed (Fig. 6 ). This sharp spectrum change reflects the transition of ordered H 2 S-γ into the disordered H 2 S-β phase. This conversion is detectable using the Raman technique only as the textural change is not instantly optically visible. The latter proceeds gradually over time (Fig. 6 ) and commences at temperature as low as −177 °C (Supplementary Table 2 ). The median temperature range for the H 2 S (γ → β) transition lies between −168.9 and −167.5 °C, whereas the median from all measurements is −168.1°C ( σ = 1.62, Supplementary Table 2 ). Upon further heating solid H 2 S (β → α) transition at about −146.4°C (B) is marked by a very slight Raman peak shift from 2549 to 2554 cm − 1 and disappearance of the tail at the higher wavenumber side. 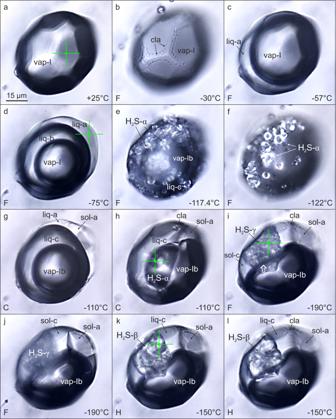Fig. 3: Microphotographs of phase transitions in CH4–H2S–CO2–N2–H2O fluid inclusion (no. P4-fi1B) in the temperature range between +25 and −190 °C, PPL, reflected light. aOne-phase gas inclusion (vap-I) at room temperature.bFormation of clathrate (cla) at the fluid inclusion corners coated by an aqueous solution.cExsolution of liquid H2S phase (liq-a).dAdvanced stage of unmixing of liquid CH4–CO2phase (liq-b).e,fInstantaneous and simultaneous crystallization of liquid H2S and liquid CO2.gNucleation of solid octahedral CO2crystal (sol-a) in the presence of liquid H2S (liq-a) by applying the cycling technique.hNucleation of a large, oval H2S solid (H2S-α) via applying the cycling technique.i,jCo-existence of polycrystalline solid H2S (H2S-γ), solid CO2octahedral crystal (sol-a), solid CH4(sol-c), clathrate (cla) and CH4-N2gas phase (vap-Ib), a prismatic H2S-γ crystal is tagged with a white arrow.k,lAppearance of solid H2S after γ → β phase transformation, visible is structure change from ordered polycrystalline to disordered “blobby” during the heating run. Symbols and abbreviations: vap-gas phases: I: CH4-H2S-CO2-N2, Ib: CH4-N2; cla-clathrate; liq-liquid phases: liq-a: H2S, liq-b: CH4–CO2, liq-c: CH4; sol-solid phases: sol-a: CO2, H2S-α,β,γ: H2S, sol-c: CH4; F-freezing run, C-cycling run, H-heating run. Green crosses mark several of Raman measurement points (see also Fig.6). During heating runs the structure of solid H 2 S phases re-organizes itself by compartmentalization of fine-grained crystals into coarser aggregates (e.g., Fig 3k, l ) in order to attain back the disordered form. Solid H 2 S-α dissolves at −98.8 °C/−99.2 °C (A/B), whereas CO 2 solid remaining in the inclusion does not preserve its octahedral habit but a rounded shape (Fig. 2l ) and melts at temperatures of −91.2 °C/−92.6 °C (A/B). After CO 2 melting the inner CH 4 –N 2 gas phase begins to expand continuously (Fig. 2m ) and partially homogenizes into a vapor phase at T h1 (L 1 L 2 V → L 2 V) = −58.4 °C/−57.8 °C (A/B, Fig. 2n ). The bubble expansion lasts until total homogenization at T h2 (L 2 V → V) = −28.6 °C/−31 °C (A/B, Fig. 2o ) is reached. The last observed change is the melting of H 2 S-rich gas hydrate (clathrate) at positive temperatures of 21.8 °C/27.5 °C (A/B, Fig. 2p ). Gas hydrates Gas hydrate crystallizes from the aqueous film containing dissolved H 2 S (Fig. 1b ) and it forms a shell surrounding the gas phase (Fig. 2b ). As a result, the H 2 S molecules become encased by the hydrogen-bonded cages in the first place and clathrate cavities are dominated by H 2 S. This is evidenced by the highest intensity of the 2592 and 2604 cm − 1 Raman peaks, which are assigned to the symmetric H–S stretching vibrations ( ν 1 ) within large cages (LC) and small cages (SC), respectively, of type I cubic lattice structure (sI) [49] . The characteristic clathrate solid (Fig. 4 ) is achieved by using a heating/freezing cycling technique, which is applied routinely in the experimental studies of gas hydrates [50] . The H 2 S-dominated clathrate (Fig. 4 ) dissociates at temperatures between +21.8 and +27.5 °C (Table 1 ), which are lower compared to the quadruple point of the H 2 O–H 2 S system ( Q 2 = + 29.55 °C [51] ). The Raman technique has also been used to identify the H 2 S-clathrate in synthetic H 2 O–H 2 S inclusions at −100 °C [52] , in natural CO 2 –H 2 S–H 2 O–S inclusions [53] and at −140 °C in natural H 2 S-bearing brine inclusions [54] . A single measurement of one individual, well-isolated clathrate crystal reveals the presence of CH 4 and minor concentrations of CO 2 and N 2 besides H 2 S molecules (Fig. 4 ). This observation suggests crystallization of H 2 S–CH 4 –CO 2 –N 2 mixed gas hydrate. The average cage occupancy ratios – θ SC / θ LC of CH 4 - and H 2 S-hydrates [49] , calculated from deconvoluted Raman spectra, are: 0.81 ( σ = 0.08) and 0.87 ( σ = 0.05), respectively. These values deviate from ratios typical of pure CH 4 and H 2 S gas hydrates [49] , [55] , probably due to incorporation of minor CO 2 and/or N 2 , which affects relative cage occupancy in the clathrate lattice. The studied clathrate crystal is most likely composed of two clusters of mixed gas hydrates, i.e., the H 2 S-dominated clathrate, which grew within the aqueous rim, and CH 4 -dominated, which developed at the water–gas interface. The N 2 molecules may occupy both small and large cavities in sI gas hydrates, as indicated by the Raman band splitting (Fig. 4a ), whereas CO 2 can occupy only large cages due to the absence of a similar peak splitting (Fig. 4 ). Nevertheless, the distribution of CO 2 and N 2 molecules between the clathrates remains ambiguous. Clathrate crystallization from the aqueous phase, containing the dissolved gas, as well as at the water–gas interface leads to depletion of available water molecules. The nucleation of gas hydrates is known to influence phase equilibria in fluid inclusions, e.g., it may decrease T m of gas components [17] . Due to the absence of dissolved/vapor H 2 O in the gas phase, the only process that may affect the gas phase density is the scavenging of gas molecules into the clathrate lattice at the water–gas interface. The water film likely has a negligible impact on the gas phase transitions as they are very consistent within FIA1 (Table 1 ), e.g., T m ’s of H 2 S ( σ = 0.05) or CH 4 ( σ = 0.3). The interaction at the aqueous film-gas phase interface has also some more limitations, e.g., the presence of dissolved H 2 S and high salinity of an aqueous solution (Fig. 1b ), which decreases the chemical potential of H 2 O resulting in a “salting out” effect [17] , [56] . Based on the above, it is apparent that only very low amounts of CO 2 and CH 4 from the gas phase have been incorporated into the clathrate lattice at low temperatures, and thus the gas phase experienced only a very minor volume change. Thereby the studied CH 4 –H 2 S–CO 2 –N 2 –H 2 O system behaves as a gas sub-system below nucleation temperature of clathrate and is interpreted as such in the following section. Applying the isochoric behavior of H 2 O-free systems to aqueous-multivolatile inclusions at low temperatures is justified as the LCEP (lower critical end-point) coincides with the critical point of the gas mixture [17] . Median compositions of the gas phase in the presence of stable clathrate at −10 °C are: 58.9 mol% CH 4 , 25.5 mol% H 2 S, 12.6 mol% CO 2 , 2.9 mol% N 2 , (FIA1), and 57.1 mol% CH 4 , 28.2 mol% H 2 S, 11.9 mol% CO 2 , 2.9 mol% N 2 (FIA2) (Supplementary Table 1 and Source Data). The CH 4 –H 2 S–CO 2 –N 2 gas system A phase diagram defining phase transitions in the multicomponent CH 4 –H 2 S–CO 2 –N 2 system has neither been experimentally nor numerically developed so far. The behavior of CH 4 –H 2 S–CO 2 mixtures, previously observed in fluid inclusions [30] , [57] , was interpreted in the frame of the CH 4 –H 2 S system [31] under the assumption that 10–20 mol% CO 2 should not significantly affect the phase boundaries. In our study the available P–T projections of phase boundaries of the CH 4 –H 2 S–CO 2 , CH 4 –H 2 S, and H 2 S systems are used to discuss the phase transitions in natural fluid inclusions. The CH 4 –H 2 S binary diagram [31] is utilized to interpret the phase behavior to −100 °C, whereas for lower temperatures, the numerically derived CH 4 –H 2 S phase diagram [35] and the phase boundaries for pure H 2 S system in the low-pressure region [40] are used (Fig. 8 ). Fluid inclusion behavior above −60 °C cannot be explained by the CH 4 –H 2 S system alone, therefore for this temperature region we use partial ternary CH 4 –H 2 S–CO 2 phase diagram [58] . Experimentally derived phase boundaries for a CH 4 –H 2 S–CO 2 system were defined only for a gas mixture with H 2 S content of 40.2 mol% [58] , which is higher than that in studied inclusions (25–28 mol%, Table 1 and Source Data), and CO 2 content of 9.87 mol%, which is close to CO 2 concentrations in the inclusions (11.9–13.3 mol%, Supplementary Table 1 ). This P–T phase diagram, based on the experimentally studied gas mixture, is, therefore, the best available approximation of the studied system at T > −83°C. Notable are three critical points in the CH 4 –H 2 S–CO 2 system: C 1 and C 2 lying along the 2-phase boundary curves, and C 3 situated on the 3-phase envelope [58] . The presence of additional gases, e.g., N 2 or CH 4 , is well known to depress the melting points in fluid inclusion gas mixtures [59] , however, we assume that N 2 quantities as low as 3 mol% would likely have a negligible effect on the phase equilibria. The trajectories followed by studied fluid inclusions (blue) during heating are shown schematically in the P–T space, in the considered diagrams (Fig. 8 ). The phase transition points (9–15) are indicated by black circles and correspond to numbers given in Table 1 . Fig. 8: Phase diagrams schematically illustrating the behavior of studied fluid inclusions in the P–T space. a Simplified phase boundaries for the system CH 4 –H 2 S [31] around critical points and the first invariant point-QP 1 with superimposed phase curves for the CH 4 –H 2 S–CO 2 system [58] (in red). b Phase boundaries for the system CH 4 -H 2 S in the lowest temperature region near the 2 nd invariant point-QP 2 point [35] and phase boundaries for pure H 2 S at low temperatures [40] . Symbols and abbreviations: upper dash-dotted line-critical curve with marked critical points for various H 2 S contents; double-dotted dashed lines-immiscibility loops for 5.25, 24.8, and 45.8 mol% H 2 S; thicker pale blue lines and arrows show schematic P–T paths followed by gas inclusions upon heating in the CH 4 –H 2 S–CO 2 and CH 4 –H 2 S systems, arrows and orange P–T path in the pure H 2 S system is followed during solid–solid phase transitions of pure H 2 S in the fluid inclusions, numbers in black circles (9–15) correspond to numbers of phase transitions during the heating cycle, which are given in Table 1 ; C 1 , C 2 , C 3 -critical points in the CH 4 –H 2 S–CO 2 system, CP–H 2 S critical point, TP–H 2 S triple point, L 2 -liquid H 2 S, L 1 -liquid CH 4 , S 2 -solid H 2 S, S 1 -solid CH 4 ; α, β, γ-solid phases of H 2 S. Full size image Cooling of fluid inclusions triggers separation of two phases at temperatures between −33 and −29.5 °C ( σ = 1.22), therefore they follow the trajectory intersecting the dew-point locus and thus enter the L 2 V 2-phase field (L 2 —liquid H 2 S, Fig. 8a ). This phase behavior is characteristic for the retrograde system as with decreasing pressure exsolution of the liquid phase takes place instead of the vapor phase. The first appearance of the liquid droplet is difficult to spot meaning that the temperature of condensation may be slightly underestimated. The P–T pathway should intersect the dew curve above the critical point C 1 , however, the temperature of the V → L 2 V transition is located below this point in the diagram. This discrepancy stems from the fact that the used phase boundaries were constructed for 40.2 mol% H 2 S. For lower H 2 S contents, alike in the studied inclusions (25–28 mol%), the dew curve would extend to lower temperatures. At temperatures between −59.6 and −57.8 °C ( σ = 0.63), closely below the critical point C 3 (−57.5 °C, where V = L 1 ), the fluid inclusion trajectory intersects the 3-phase L 1 L 2 V boundary emanating from the C 3 point (L 1 —liquid CH 4 , Fig. 8a ). It is manifested by the separation of a third phase in the inclusion and marks the exsolution of a first drop of methane condensate. Under the optical microscope the newly formed phase appears vapor-like (Figs. 2d and 3d ), probably due to the very close proximity of the C 3 . Since fluid inclusions contain two immiscible liquid phases and a vapor they follow the path along the L 1 L 2 V phase boundary and at about −122 °C reach the invariant point: QP 1 (Fig. 8a ). At the QP 1 , in the CH 4 –H 2 S system four phases co-exist: solid H 2 S-α, liquid H 2 S, liquid CH 4 and a vapor [31] . In the analyzed system, the simultaneous and instant solidification of H 2 S and CO 2 (Figs. 2e and 3e ) is observed, thus in the 3-component CH 4 –H 2 S–CO 2 system five phases co-exist in equilibrium at the invariant quintuple point-QP 1 : H 2 S solid, CO 2 solid, CH 4 liquid, H 2 S + CO 2 liquid, and a vapor. If N 2 component is considered the number of phases at equilibrium remains the same, however, the QP 1 is converted into a univariant curve in the P–T space. The solidification of H 2 S–CO 2 is subject to metastability as the measurements of the same inclusion yield a range of temperatures, and similar variability is also reflected by measured FIA1 ( σ = 4.58, Table 1 ). The freezing temperatures ( T n ) are relatively lower compared to melting temperatures ( T m ) of H 2 S or CO 2 (Table 1 ), which requires supercooling to nucleate solids. Precipitation of pure solid H 2 S-α in the presence of pure solid CO 2 increases the temperature of the QP 1 to between −107 and −104 °C (Table 1 ), when the cycling technique is applied. Contemporaneous freezing of H 2 S and CO 2 is typically observed in binary H 2 S–CO 2 systems at an eutectic temperature of −95.6 °C, where the S CO2 LV and S H2S LV triple-point loci converge at the quadruple point [32] . The phase behavior, observed in the studied fluid inclusions, can thus be explained by an overlap of quadruple points of the binary CH 4 –H 2 S and H 2 S–CO 2 systems. Moreover, the H 2 S-CO 2 freezing point temperatures between −125.9 and −114.9 °C (Table 1 ), measured in the CH 4 –H 2 S–CO 2 –N 2 inclusion gas phase with 11.9–13.3 mol% CO 2 (in the presence of clathrate, Source Data), are much lower compared to the eutectic temperature for binary H 2 S–CO 2 gas mixtures. According to experimental studies, the latter gas mixtures with <12.5 mol% CO 2 , follow triple point equilibria with solid H 2 S in the binary systems and do not represent eutectic mixtures [32] . Therefore, our study shows that the presence of CH 4 gas has a significant impact on the phase behavior of H 2 S–CO 2 gases in studied natural fluid inclusions. From the QP 1 point onwards fluid inclusions follow the S 2 L 1 V phase boundary and after intersecting the second quintuple point-QP 2 at temperatures between −188 and −185.3 °C ( σ = 0.97), the S 1 S 2 V curve becomes a path (Fig. 8b ). At the QP 2 two solids: CH 4 (S 1 ) and H 2 S (S 2 ), liquid CH 4 and vapor phases are co-existing in equilibrium in the CH 4 –H 2 S system. The position of the QP 2 point in this binary system is determined by SLV equation of state since experimental data are lacking [35] . In the CH 4 –H 2 S–CO 2 system, five phases co-exist at QP 2 : H 2 S solid, CO 2 solid, CH 4 solid, CH 4 liquid, and a vapor. Our study shows that both solidification and melting of methane progress gradually over a temperature interval as the liquid/solid methane phase boundary has been clearly observed (Fig. 2h, j ). During the latter phase transition five phases: S 1 S 2 L 1 V, where S 2 stands for both H 2 S and CO 2 solids, are co-existing (Fig. 2h, j ). Comparison of T n and T m values of CH 4 , measured in the inclusion gas mixtures (Table 1 ), reveals that only slight supercooling is required to nucleate solid CH 4 and it is achievable using liquid N 2 coolant during microthermometry runs. Melting of methane (point 9 in Fig. 8b ) occurs at T m between −186.3 and −184.1 °C, which are very consistent ( σ = 0.3, Table 1 ) and lie slightly below the triple point of a pure CH 4 system (−182.48 °C) and a quadruple point-QP 2 of the CH 4 –H 2 S system (−182.4 °C [35] ). The melting temperatures of H 2 S-α solid (point 12 in Fig. 8a ) within FIA1 (from −98.9 to -98.8 °C) show extremely low variability ( σ = 0.05), which corresponds to stable H 2 S contents in the inclusions (Table 1 ). Solid CO 2 melts (point 13 in Fig. 8a ) at temperatures −91.2°C/−92.6 °C (A/B). Elevated standard deviation ( σ = 1.14) for T m (CO 2 ) may be due to slight compositional variation in the inclusions (11.9–13.3 mol% CO 2 ) or due to difficulties in T m observations, which stem from a small difference in refractive indices between the liquid phase and very small CO 2 crystals. Melting of all three solids: CH 4 , H 2 S, and CO 2 proceeds over temperature intervals, which is characteristic of multicomponent gas systems [17] , [60] . The median T m values (FIA1): −184.3 °C (CH 4 ), −98.9 °C (H 2 S) and −91.9 °C (CO 2 ) are depressed compared to temperatures of melting points of the relative unary systems, i.e., −182.5 °C (CH 4 ), −85.5 °C (H 2 S), and −56.6 °C (CO 2 ). This implies that such melting behavior is not only typical for multivolatile H 2 S-free systems [17] , but also for H 2 S-rich gas mixtures. At the point, where the last solid-phase melts, the fluid inclusions follow back the L 1 L 2 V curve (point 13 in Fig. 8a ). The first partial homogenization T h1 (L 1 L 2 V → L 2 V) takes place in a similar temperature interval from −59.8 to −57.6 °C ( σ = 0.78, point 14 in Fig. 8a ) as the relative opposite phase transition during cooling (no. 3 in Table 1 ). This enforces the inclusions to enter the 2-phase L 2 V field (Fig. 8a ) until the homogenization to the vapor (L 2 V → V), through a dew-point transition, takes place at temperatures between −32.5 and −28.6 °C ( σ = 1.31). During the latter transition 2-phase fluid inclusions (L 2 V) follow back the trajectory intersecting the dew-point locus (point 15 in Fig. 8 ) and enter the vapor 1-phase field (Fig. 8a ). H 2 S solid–solid transitions in fluid inclusions The observation of low-temperature H 2 S solid–solid transitions (α ↔ β ↔ γ) in natural fluid inclusions requires consideration of new phase boundaries: S 2α S 2β L 1 V and S 2β S 2γ L 1 V, and their influence on the CH 4 –H 2 S–CO 2 –N 2 system. The experimentally determined solid–solid transitions of pure H 2 S occur at temperatures of −169.55 and −146.95 °C [40] , [42] , [61] , which are above the QP 2 point of the CH 4 –H 2 S system (Fig. 8b ). The temperature range of the H 2 S (β → γ) transformations measured in the studied inclusions indicate that the above expected equilibrium temperatures are not sustained along the cooling pathway. In order to nucleate H 2 S-γ undercooling or maintaining a constant temperature for a period of time is required, which indicates metastable behavior or kinetics problems. The measured temperatures of the H 2 S(γ → β) transition in the studied inclusion are oscillating around an average of −168.1 °C (point 10 in Fig. 8b , Supplementary Table 2 ), which is slightly higher compared to the corresponding value for a pure H 2 S system (−169.55 °C). This may be related to pressure as the P–T diagram for phase transitions of pure (99.5%) solid H 2 S, at low pressures, shows that temperatures of solid–solid transitions increase with increasing pressures [40] (Fig. 8b ). The H 2 S (γ → β) transition is peculiar as after commencement it gradually proceeds even without temperature increase (on hold) with only the laser on, irrespectively of the laser power used. The temperatures of −147 and −146.4 °C for the solid H 2 S(β → α) transitions in the studied fluid inclusion (point 11 in Fig. 8b ) are in a very good agreement with the experimentally derived temperature of −146.95 °C (Fig. 8b ). According to numerical modeling [35] allotropic behavior of solid H 2 S does not affect significantly the overall solid-fluid equilibria of the CH 4 –H 2 S mixture. Instead, the modeling has shown that in the CH 4 –H 2 S system the temperatures of solid–solid H 2 S transitions are depressed relative to corresponding temperatures in pure H 2 S system [35] . This hypothesis is not consistent with H 2 S(γ ↔ β ↔ α) transitions temperatures in the natural fluid inclusions studied here and shows that the presence of CH 4 –CO 2 gas affects solid–solid H 2 S phase equilibria in gas mixtures. Experimental studies of laboratory-grown H 2 S crystals has shown that the solid H 2 S(γ → β) transition is attributed to a decrease in the dielectric constant, whereas the H 2 S(β → α) transition is ascribed to orientational ordering relative to the rotational vibrations of the hydrogen atoms [61] . During the higher temperature transition, the crystal structure of both phases (α, β) of fluid inclusion H 2 S remains disordered, which is expressed by broad bands observed in the stretching region of the Raman spectrum (Fig. 6 ) and “blobby” appearance under the optical microscope (Figs. 2g and 3e, f, h, l ). The number of peaks and their bandwidths shifts, at the point of the lowest temperature transformation (Fig. 6 ), imply structural modifications of solid H 2 S (Fig. 3i ). The crystalline H 2 S-γ solid, which nucleates in natural fluid inclusions, shows peaks at wavenumbers (Fig. 7 ) very similar to those detected by an experimental study of purified H 2 S gas [39] . Microscopic observations during low-temperature runs unambiguously show a structural change to a polycrystalline aggregate with in-situ growing prismatic crystals (Fig. 3i ) and confirm the crystalline nature of the studied H 2 S-γ phase. Two crystal systems, orthorhombic or tetragonal, were proposed for solid H 2 S-γ phase [39] , [41] . Our study clearly shows that the protracted structural transformations do not immediately follow up the low-temperature phase transitions detected by Raman spectroscopic analyses. Spectral features of complex gas mixtures Systematic shifts of Raman peak positions are observed for all inclusion gas species during the measurements. They are most pronounced for H 2 S and CH 4 due to their high concentrations in the studied gas-rich inclusions (Figs. 5 and 6 ). Experimental studies have shown that changes in pressure, temperature and density of a single gas component as well as CH 4 –CO 2 gas mixtures have an influence on the Raman peak positions [62] , [63] , [64] . Modifications of gas peak positions in H 2 S-bearing ternary, as well as any more complex gas mixtures, have not been studied so far. Our results show that the Raman band positions are shifted to higher wavenumbers for more volatile components and to lower wavenumbers for less volatile components, relative to the original peak positions of the gas mixture at room temperature (Fig. 5 ). This tendency is also marked by systematic trends in diagrams illustrating H 2 S and CH 4 band positions (cm − 1 ) versus temperature (Fig. 9 and Source Data). It is observed that the FWHM (full width at half maximum) of the peaks of gaseous, liquid, and solid CH 4 phases, which exsolved from the CH 4 -H 2 S-CO 2 -N 2 gas mixture, consistently decrease with decreasing temperatures (Fig. 5 ). The above-mentioned features reflect well differential partitioning between the co-existing phases in an individual inclusion upon cooling, which is the strongest at the lowest recorded temperatures of about −190 °C (Fig. 9 ). The observations also reveal that gases of the highest volatility, i.e., N 2 and CH 4 , partition into the inner vapor phase, whereas CO 2 and H 2 S partition into the outer liquid phases. Similar distribution of gaseous components between the phases has been described for binary gas mixtures [17] . Our study shows that the composition of the gas mixture affects the wavenumbers of its gas components, e.g., CH 4 peak measured in the gas mixture at room temperature is positioned at 2911 cm − 1 , whereas at −190 °C it shifts to 2917 cm − 1 (Fig. 9 ), which is the wavenumber typical of pure CH 4 gas. The band position downshifts can also be indirectly related to the density difference between gas, liquid, and solid physical states of the inclusion components, i.e., solid H 2 S or CH 4 show shifts to the lowest wavenumbers: 2522 and 2904 cm − 1 , respectively (Fig. 9 ). Fig. 9: Diagrams showing the relationship between temperature and Raman band wavenumbers. a Shifts in peak positions of H 2 S vapor, liquid, and solid (α, β, γ) phases with decreasing temperature. The measurements were recorded in 10 °C increments. b Shifts in band positions of vapor, liquid and solid CH 4 with decreasing temperature. The measurements were recorded in 30 °C increments. Both H 2 S and CH 4 show similar trends, namely Raman peak positions of volatile phases shift towards higher wavenumbers, whereas less volatile components reveal opposite tendency. This discrepancy reflects differential partitioning between co-existing phases. The data were collected from one individual fluid inclusion (no. P1a-fi10) during the heating run. The peak positions were calibrated using neon emission lines. See also Source Data file. Full size image Experimental models and databases We report on new fluid inclusion-derived temperature, compositional and spectroscopic data on a multicomponent CH 4 –H 2 S–CO 2 –N 2 –H 2 O system. The results of our study are helpful not only for the interpretation of phase equilibria observed in fluid inclusion gas mixtures but also can be used as a guide for future experimental studies of fluids utilizing, e.g., synthetic fluid inclusions, fused-silica optical cells, or silica capillary tubes. Such studies are necessary to construct the unified complete topology of the C–O–H–N–S chemical system, which is required to improve understanding of the phase equilibria [29] . Such purely experimental results cannot ideally reproduce natural systems, hence data from natural fluid inclusion gas–H 2 O mixtures are complementary and can be used for validation and models refinement. Detailed characterization of phase transition (α ↔ β ↔ γ) temperatures, structural transformations and spectral features of different solid H 2 S phases, in natural fluid inclusions, contribute to the advancement of scientific knowledge about the nature of the H 2 S solid–solid-phase equilibria. Our study shows that the band wavenumbers of gas components in the natural CH 4 –H 2 S–CO 2 –N 2 gas mixtures differ from the standard Raman shifts (Δ ν in cm − 1 ) known from the Raman databases, and thus have a substantial impact on interpretation of literature data. It has been shown here that gas peak modifications in ternary H 2 S-bearing and more complex gas mixtures depend on their compositions as well as on relative density differences arising from differential partitioning of the gas mixture components in a closed system. These findings constitute new and valuable insights into the behavior of individual gases in multi-gas mixtures in natural fluid systems. Hydrocarbon and mineral systems The improved understanding of complex gas–H 2 O systems is a prerequisite for more accurate reconstruction of the P–T conditions in hydrocarbon and mineralizing fluid systems in the geological record. The P–T information obtained from studies of fluid inclusions hosted in cements and facture-filling minerals provide means for the reconstruction of multiple fluid and gas migration events in hydrocarbon reservoirs and contribute, e.g., to enhancement of gas accumulation models [22] . The migration of geological fluids, carrying reduced sulfur species (e.g. H 2 S, HS − ), has a paramount control on the deposition of hydrothermal ore deposits. In evaporitic diagenetic environments of sedimentary basins, hydrocarbon and ore mineral systems are often closely linked [10] . In cases where the circulating basinal brines or formation waters are devoid of sufficient metal content to form sulfide ores, by mixing with H 2 S-rich fluids, the latter may accumulate in gas/petroleum traps within sedimentary sequences and may pose risks for hydrocarbon exploration and environmental hazards. Constraining the geological time frames and depth intervals of thermochemical sulfate reduction (TSR) [8] is also of high importance as it produces H 2 S and CO 2 , which contaminate hydrocarbon reservoirs [6] , [65] , [66] . Microthermometric studies of CH 4 –H 2 S–CO 2 –N 2 fluid inclusion gas mixtures allow the prediction of freezing points of H 2 S and CO 2 . Our study indicates that at low temperatures of about −122 °C (Table 1 ), the H 2 S-CO 2 gases in analyzed gas inclusions show very unique behavior of contemporaneous freezing, which is likely linked to the subordinate amounts of CO 2 (11.9–13.3 mol%). Therefore, CH 4 -rich gas mixtures have a potential for relatively efficient purification to commercial quality grades by using, e.g., low-temperature distillation process [38] . However, the disposal of resulting by-products (H 2 S, CO 2 ) rises substantial environmental concerns as geochemical behavior of these gases in various deep geological formations is not yet well constrained [67] . Our study demonstrates that gas-rich CH 4 –H 2 S–CO 2 –N 2 –H 2 O fluid inclusions offer an excellent opportunity to study the formation of complex natural gas hydrates in a closed system. Due to global warming, there is an increasing interest in understanding the behavior of natural gas hydrates that were discovered in deep-sea environments and permafrost regions [49] . The formation mechanisms, as well as structural and compositional heterogeneities of the complex/mixed natural clathrate crystals, are not yet fully understood [50] , [51] . Comparison of experimental simulations of synthetic gas hydrates with systematic studies of natural gas–H 2 O inclusions mixtures provides means for a better understanding of the kinetics and thermodynamics of clathrates formation and dissociation. Such knowledge is relevant to investigations of synergies between CH 4 -gas hydrates and climate change on a global scale [68] . Extraterrestrial systems Low-temperature systems, which are a prerequisite for solid–solid H 2 S transitions do not exist in terrestrial environments, but they persist on ice planets such as Uranus and Neptune [12] , [13] . Recent studies evidenced the presence of gaseous H 2 S above the cloud deck of Uranus, which led to the conclusion that H 2 S ice is a major constituent of main clouds at 1.2–3 bar [12] . Similarly, the H 2 S ice is considered to be a prime constituent of Neptune’s main clouds at pressures of 2.5-3.5 bar [13] . At extremely low temperatures (from ca. −220 °C [11] to −153.7 °C [12] ), at various depth levels in the ice giants atmosphere’s, there is thus a high likelihood that H 2 S ice cloud decks exist in different temperature-dependent solid states. This, in turn, may potentially have an influence on the atmospheric dynamics of the ice planets. Recent studies point also towards differences in the distribution of H 2 S ice and CH 4 , between polar and equatorial regions of the Uranus’s atmosphere, which yet require explanation [12] . The latter could provide valuable insights into the atmospheric dynamics of the enigmatic ice giants [69] . Possible future exploratory missions to the ice planets would benefit from having a Raman spectrometer on board, which allows identification of possible perturbations caused by distinct H 2 S solid states and constraining distribution of H 2 S ice and associated gases at low temperatures. A miniaturized Raman spectrometer has been used, e.g., in a mission to Mars [70] . Microthermometry For this study, we used fracture-filling fluorite mineralization, hosted by Upper Permian Zechstein Ca 2 carbonate from the Southern Permian Basin, Germany. The drill core sample originates from a depth of ca. 3.8 km from well PB-20 situated at the border of the Pompeckj Block and the northern flank of the Lower Saxony Basin [8] . The translucent coarse fluorite crystals, selected for analyses, host abundant CH 4 –H 2 S–CO 2 –N 2 –H 2 O fluid inclusions (Fig. 1 and Table 1 ). Doubly-polished fluorite chips (~8 × 8 mm) with a thickness of 180 μm were used for analyses. Microthermometric and laser Raman spectroscopic measurements were performed at the GFZ Potsdam, Germany. Microthermometry and observations of phase changes in gas-rich inclusions were conducted using a Linkam heating/freezing stage (THMS600 system) that allows observations of phase transitions in fluid inclusions in the temperature range between −195 and 600 °C. The heating/freezing system was calibrated using SynFlinc synthetic fluid inclusion standards: CO 2 and pure H 2 O for melting temperatures of CO 2 and ice, respectively as well as critical homogenization temperature of pure H 2 O. Temperatures were recorded using Linksys 32 software with reproducibility of ±0.1 °C. Imaging during the microthermometry runs was performed using a digital QICAM FAST1394 camera attached to an Olympus BX53M microscope and the Q-Capture Pro 7 software was used for image acquisition. Raman spectroscopy combined with microthermometry Laser Raman spectroscopy coupled with microthermometric experiments was utilized to examine phase changes and solid phases formed at low temperatures. Measurements were performed using the Linkam THMS600 system equipped with LNP95 nitrogen cooling pump, T95 temperature controller, and a stage with a silver heating/freezing block and a PT100 platinum sensor. The Linkam heating-freezing stage was calibrated using the synthetic CO 2 and H 2 O fluid inclusion standards, provided by SynFlinc, prior to Raman spectroscopic analyses. The temperatures were recorded, in a range between −192 and +35°C, using a Linksys 32 software with reproducibility of ±0.1 °C. Heating/freezing rates during measurements of the phase transitions were 4 °C/min or/and 10 °C/min, whereas in between the phase transitions the rates were 20–30 °C/min. The vibrational spectra of phases in gas-rich inclusions during freezing-heating runs were measured using a LabRAM HR Evolution Raman micro-probe supplied by Horiba Scientific. The system is equipped with a dispersive Raman spectrometer with focal length of 800 mm, the frequency-doubled Nd:YAG solid-state green laser source with an excitation radiation of 532 nm and output power of 100 mW (max. ~48 mW at the sample surface), edge filters, and a CCD detector. A grating of 1800 grooves/mm and confocal hole of 100 µm were used, and the spectral resolution was 1 cm − 1 . Most measurements (when not indicated otherwise) were performed using a neutral density filter, which reduces the output laser power at the sample to 50% (~24 mW) to avoid frequent “out of range” high intensity CH 4 peaks with artificially cut tops. Internal calibration has been performed using a silicon standard (520 cm − 1 ). A neon lamp attached to the Linkam stage was used for a wavenumber calibration. The spectra of Ne emission lines were collected simultaneously with each peak position measurement. The reference Ne emission lines used for the wavenumber calibration of H 2 S were: 2389, 2708 cm − 1 , and of CH 4 : 2835, 3006 cm − 1 . The peak positions, corrected for instrumental drift, were calculated using the measured wavenumbers of H 2 S, CH 4 (symmetric stretching ν 1 vibrational modes), Ne lines, and applying the linear interpolation equation [71] . The average standard error for peak position measurements at room temperature, based on 8 measurements (2 inclusions measured 4×), was 0.02 cm − 1 for CH 4 and 0.01 cm − 1 for H 2 S. The uncertainty of the peak wavenumber measurements was ±1 cm − 1 for all gas components [64] . The Raman spectrometer is adapted to an Olympus BXFM optical microscope, which is equipped with 50× (NA = 0.5) long working distance objective, reflected and transmitted light sources, and a VIS Camera. This setup enables optical investigation of phase transitions in fluid inclusions as well as photographic documentation during the combined experiments. The Raman spectra were acquired by focusing the laser beam on analyzed phases, in the spectral range between 250 and 4500 cm − 1 and with 2 × 20s acquisition time. The spectra were processed using LabSpec software (ver. 6.4.4.16). The linear baseline correction and the Gaussian–Lorentzian peak-fitting function were used for processing and deconvolution of the Raman spectra. The concentrations of the aqueous solution (molar fractions) were measured in homogenized inclusion fluid in a temperature range between 160 and 170 °C [45] . 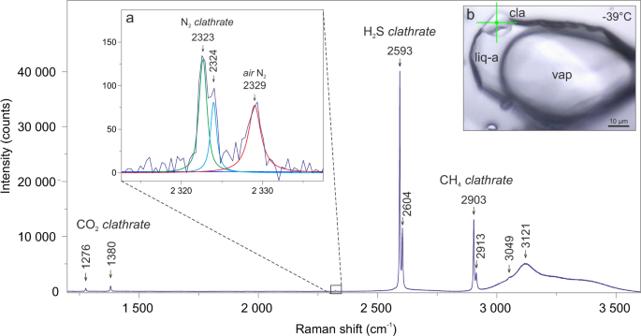Fig. 4: Raman spectrum of natural clathrate in CH4-H2S-CO2-N2-H2O fluid inclusion (no. P1a-fi10) at −39 °C. An individual measurement records complex clathrate phase/s containing H2S, CH4and minor CO2, N2molecules. Additional Raman peaks at 3049 and 3121 cm−1, present in the O-H stretching spectral region, are assigned to a molecular vibration of CH4occluded in the hydrate lattice49and ice, respectively.aThe inset shows low-intensity Raman bands corresponding to N–N stretching vibrations in N2-gas hydrate48and air N2.bMicrophotograph of the analyzed clathrate solid in gas-rich inclusion. Symbols: vap-CH4–H2S–CO2–N2gas phase, cla-measured clathrate phase, liq-a-liquid H2S phase, the measurement point is marked with a green cross. The spectrum was acquired with 100% laser power. Molar fractions of gases in the gas mixtures trapped in inclusions were derived from the ratios of the Raman peak areas and applying the formula based on Placzek’s polarizability theory [23] , [29] , [62] . 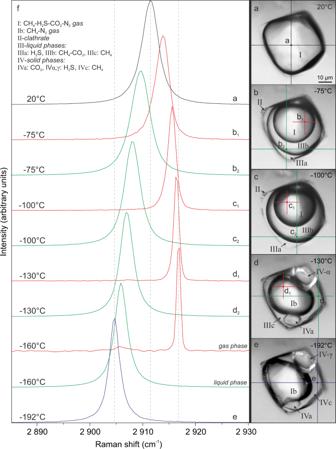Fig. 5: Raman spectra of symmetric stretching (ν1) region of CH4gas in a natural CH4–H2S–CO2–N2–H2O fluid inclusion gas mixture (no. P1-fi1A) at low temperatures. a–eMicrophotographs of measured individual phases in analyzed gas-rich inclusion.fSequence of Raman spectra showing that with decreasing temperature Raman peak positions of the exsolved liquid and gas methane shift to lower and higher wavenumbers, respectively. This is a result of relative density increase/decrease during differential partitioning between co-existing phases. The FWHM of the Raman peaks also decrease with decreasing temperatures. Symbols: I: CH4–H2S–CO2–N2gas, Ib: CH4–N2gas, II-clathrate, III-liquid phases: IIIa: H2S, IIIb: CH4–CO2, IIIc: CH4, IV-solid phases: IVa: CO2, IVα,γ: H2S, IVc: CH4, measurement points of different phases are marked with large and small crosses. 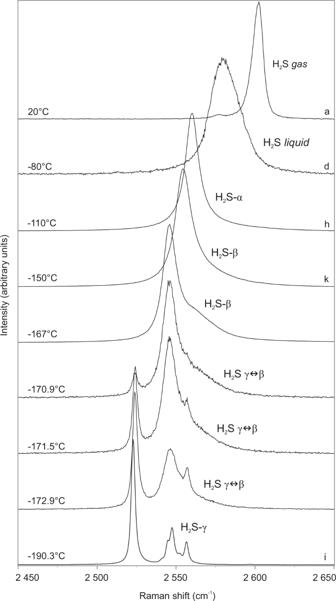Fig. 6: Raman spectra of the stretching region of H2S in a natural CH4–H2S–CO2–N2–H2O fluid inclusion (no. P4-fi1B) at low temperatures. A density-related shift in Raman peak positions to lower wavenumbers with decreasing temperature is observed for different physical states of H2S. The measurement points (a, d, h, k, i) are indicated by green crosses in the Fig.3. The solid H2S (γ ↔ β) phase transition is marked by intensity decrease of the characteristic peak of the β-phase and the progressive emergence of the sharp γ-phase peak at the lower wavenumber (2523 cm−1) and its subsequent intensity increase. The solid H2S (γ ↔ β) phase transition was recorded during real-time measurements. 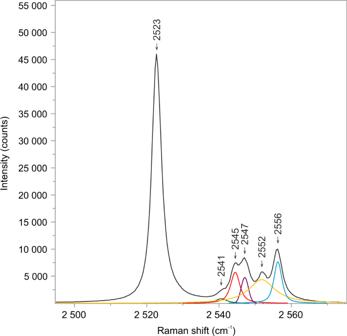Fig. 7: Raman spectrum of solid H2S-γ in a natural CH4–H2S–CO2–N2–H2O fluid inclusion (no. P4-fi1B). Six characteristic peaks are observed in the H–S spectral region at −191 °C. Five overlapping peaks have been deconvolved into separate bands and fitted using the Gaussian–Lorentzian peak-fitting function. The spectrum was acquired with 100% laser power. 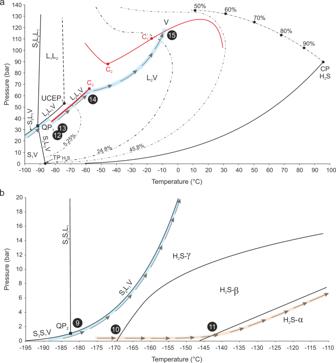Fig. 8: Phase diagrams schematically illustrating the behavior of studied fluid inclusions in the P–T space. aSimplified phase boundaries for the system CH4–H2S31around critical points and the first invariant point-QP1with superimposed phase curves for the CH4–H2S–CO2system58(in red).bPhase boundaries for the system CH4-H2S in the lowest temperature region near the 2ndinvariant point-QP2point35and phase boundaries for pure H2S at low temperatures40. Symbols and abbreviations: upper dash-dotted line-critical curve with marked critical points for various H2S contents; double-dotted dashed lines-immiscibility loops for 5.25, 24.8, and 45.8 mol% H2S; thicker pale blue lines and arrows show schematic P–T paths followed by gas inclusions upon heating in the CH4–H2S–CO2and CH4–H2S systems, arrows and orange P–T path in the pure H2S system is followed during solid–solid phase transitions of pure H2S in the fluid inclusions, numbers in black circles (9–15) correspond to numbers of phase transitions during the heating cycle, which are given in Table1; C1, C2, C3-critical points in the CH4–H2S–CO2system, CP–H2S critical point, TP–H2S triple point, L2-liquid H2S, L1-liquid CH4, S2-solid H2S, S1-solid CH4; α, β, γ-solid phases of H2S. 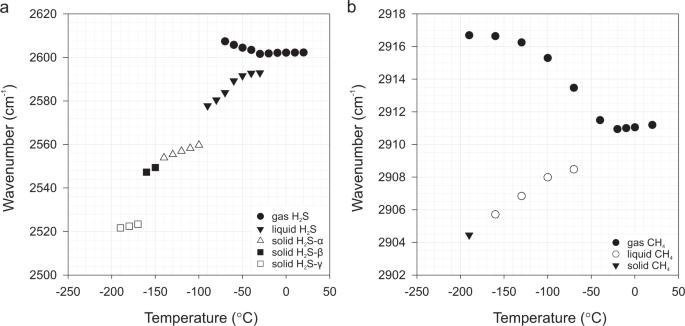Fig. 9: Diagrams showing the relationship between temperature and Raman band wavenumbers. aShifts in peak positions of H2S vapor, liquid, and solid (α, β, γ) phases with decreasing temperature. The measurements were recorded in 10 °C increments.bShifts in band positions of vapor, liquid and solid CH4with decreasing temperature. The measurements were recorded in 30 °C increments. Both H2S and CH4show similar trends, namely Raman peak positions of volatile phases shift towards higher wavenumbers, whereas less volatile components reveal opposite tendency. This discrepancy reflects differential partitioning between co-existing phases. The data were collected from one individual fluid inclusion (no. P1a-fi10) during the heating run. The peak positions were calibrated using neon emission lines. See also Source Data file. The average standard error for estimation of mole fractions, based on 14 measurements (2 inclusions measured 7×), was 0.001 cm − 1 for each gas component.